Ultrafast charge localization in a stripe-phase nickelate Self-organized electronically ordered phases are a recurring feature in correlated materials, resulting in, for example, fluctuating charge stripes whose role in high- T C superconductivity is under debate. However, the relevant cause–effect relations between real-space charge correlations and low-energy excitations remain hidden in time-averaged studies. Here we reveal ultrafast charge localization and lattice vibrational coupling as dynamic precursors of stripe formation in the model compound La 1.75 Sr 0.25 NiO 4 , using ultrafast and equilibrium mid-infrared spectroscopy. The opening of a pseudogap at a crossover temperature T * far above long-range stripe formation establishes the onset of electronic localization, which is accompanied by an enhanced Fano asymmetry of Ni-O stretch vibrations. Ultrafast excitation triggers a sub-picosecond dynamics exposing the synchronous modulation of electron–phonon coupling and charge localization. These results illuminate the role of localization in forming the pseudogap in nickelates, opening a path to understanding this mysterious phase in a broad class of complex oxides. The self-organized segregation of charges into atomic-scale patterns is an expression of the interplay between competing interactions that governs the physics of correlated transition metal oxides [1] , [2] . In high- T C superconductors, recent studies have observed fluctuating charge order above T C [3] , [4] , [5] , [6] . This raises questions about the causal relation between dynamical stripe fluctuations and the yet unexplained pseudogap phase [3] , [5] , [7] and encourages studies of real-space charge correlations on short length and timescales. A particularly intriguing model system to explore stripe physics is the nickelate compound La 2− x Sr x NiO 4 (LSNO), which is isostructural to cuprates yet exhibits real-space charge and spin stripes without superconductivity at relevant doping levels [8] , [9] . In addition, the nickel oxide class of materials has recently attracted growing attention because of novel applications in oxide electronics [10] , [11] . The electromagnetic response of nickelates is characterized by a mid-infrared (mid-IR) gap in the optical conductivity [12] , [13] , [14] , [15] , [16] along with strongly temperature-dependent lattice vibrations [15] , [17] . However, the relationship between stripe formation and these excitations remains unresolved, with the optical gap attributed alternatively to static charge order, fluctuating stripes or small polarons driven by strong lattice coupling [12] , [13] , [14] , [15] , [16] , [17] . In this context, ultrafast broadband spectroscopy provides tools to clarify the coupling between degrees of freedom in correlated systems by probing the time evolution of intrinsic excitations after sudden perturbation [18] , [19] , [20] , [21] . The ability of ultrafast optical pulses to suppress the long-range stripe order was, moreover, recently demonstrated in nickelates via time-resolved resonant X-ray diffraction [22] , [23] . Here we combine broadband ultrafast mid-IR spectroscopy with equilibrium optical and X-ray diffraction (XRD) studies to explore the low-energy excitations of a stripe-phase nickelate and their coupling in space and time. By investigating a lightly doped LSNO sample ( x =0.25), we identify the mid-IR optical gap as a pseudogap feature, clearly distinct from long-range stripe ordering. We show that the pseudogap arises from electronic localization and is accompanied by a peculiar Fano asymmetry of the Ni-O stretching mode. Ultrafast photo-induced delocalization of holes triggers a strong suppression of this Fano asymmetry, whose swift recovery closely mimics the pseudogap (localization) dynamics. These results suggest the strong and rapid dependence of electron–phonon coupling on the local charge arrangement and identify electronic localization as a dynamic precursor to stripe formation. 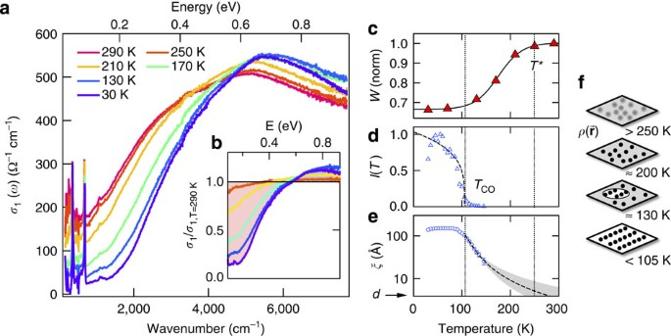Figure 1: Equilibrium optical conductivity and charge-order correlations. (a), In-plane optical conductivityσ1(ω) of LSNO (x=0.25) at different temperatures, and (b), data normalized to theT=290 K room temperature conductivity. The shaded area indicates the difference between the normalized conductivities at room temperature and at 30 K. (c) Temperature dependence of spectral weight below 0.6 eV, revealing a smooth crossover belowT*≈250 K. Line: guide to the eyes. (d,e) Intensity and in-plane correlation length obtained from XRD from the charge-ordering superlattice atq=(0.554,0,1). The correlation length is plotted on a log scale to elucidate the high-temperature trend. Dashed lines are the fits with critical scaling laws25for the intensityI(T)[(Tco−T)/Tco]2βwithβ=0.17±0.07 and correlation lengthξ(T)[(T−Tco)/Tco]−vwithv=1.47±0.15, where the statistical error represents the 95% confidence interval in extracting the fitting parameters. Within the experimental accuracy, the value of the exponentvis compatible with a 2D percolative model25, wherev=1.32. Shaded area: critical model extrapolation with twice the error bars on the fitting parameters to include possible deviations from the critical scaling law at higher temperatures. (f) Sketch of real-space charge density distribution in the Ni-O plane at different temperatures. Equilibrium optical conductivity and XRD The La 1.75 Sr 0.25 NiO 4 single crystal investigated by us exhibits long-range charge stripes below the charge-ordering temperature T CO ≈105 K, accompanied by incommensurate spin order below ≈90 K. Figure 1a shows the real part of the equilibrium optical conductivity σ ( ω ) at different sample temperatures, where the optical polarization is aligned along the ab plane to probe the charge dynamics within the Ni-O sheets. These spectra were obtained by Fourier-transform IR spectroscopy measurements of the sample reflectivity R ( ω ) between ≈10 meV–1 eV, which was converted into the complex-valued conductivity σ ( ω )= σ 1 ( ω )+ i σ 2 ( ω ) using a Kramers–Kronig constrained variational method (see Kuzmenko [24] ). With decreasing temperature, we observe a depletion of the low-frequency conductivity ( Fig. 1a ), as spectral weight is progressively removed and redistributed into the energy region above 0.6 eV. The transfer involves almost 80% of the spectral weight below 250 meV, as evident from the normalized conductivity in Fig. 1b . It can be quantitatively analysed by the low-energy spectral weight , where the cutoff frequency ω c ≡0.6 eV is chosen to coincide with the nearly isosbestic point in σ 1 ( ω ). Figure 1: Equilibrium optical conductivity and charge-order correlations. ( a ), In-plane optical conductivity σ 1 ( ω ) of LSNO ( x =0.25) at different temperatures, and ( b ), data normalized to the T =290 K room temperature conductivity. The shaded area indicates the difference between the normalized conductivities at room temperature and at 30 K. ( c ) Temperature dependence of spectral weight below 0.6 eV, revealing a smooth crossover below T *≈250 K. Line: guide to the eyes. ( d , e ) Intensity and in-plane correlation length obtained from XRD from the charge-ordering superlattice at q =(0.554,0,1). The correlation length is plotted on a log scale to elucidate the high-temperature trend. Dashed lines are the fits with critical scaling laws [25] for the intensity I ( T ) [( T co − T )/ T co ] 2 β with β =0.17±0.07 and correlation length ξ ( T ) [( T − T co )/ T co ] − v with v =1.47±0.15, where the statistical error represents the 95% confidence interval in extracting the fitting parameters. Within the experimental accuracy, the value of the exponent v is compatible with a 2D percolative model [25] , where v =1.32. Shaded area: critical model extrapolation with twice the error bars on the fitting parameters to include possible deviations from the critical scaling law at higher temperatures. ( f ) Sketch of real-space charge density distribution in the Ni-O plane at different temperatures. Full size image The dramatic changes in σ 1 ( ω ) indicate the loss of itinerancy by hole carriers concurrent with the opening of a low-temperature mid-IR gap. However, the spectral weight transfer W ( T ) lacks a sharp transition at the ordering temperature T CO ( Fig. 1c ). Instead, we observe a smooth crossover starting around a temperature T *≈250 K much higher than T CO . For comparison, Fig. 1d shows the intensity of X-ray diffraction resonant to the Ni L 3 -edge from our sample at the charge-order wave vector [22] . It drops quickly upon approaching T CO and follows the known two-dimensional (2D) critical scaling (solid line, Fig. 1d ), reflecting the disappearance of long-range stripes [25] . The high onset temperature T * of the spectral weight transfer in σ 1 ( ω ) contrasts with the expectation of a charge-order gap opening at T CO because of breaking of the translational symmetry. The features in σ 1 ( ω ) thus instead represent a pseudogap in the mid-IR charge transport, governed by microscopic physics beyond the formation of long-range stripes. Our study of a lightly doped nickelate with a relatively low T CO allows for a clear separation of these two temperature scales. Importantly, however, in XRD a residual signal also persists beyond the transition at T CO , which indicates the presence of charge-stripe fluctuations above T CO . The correlation length ξ of the fluctuations obtained from the width of the diffraction peak is shown in Fig. 1e : it rapidly shortens as the temperature increases above T CO . Extrapolating this trend above T CO with a critical scaling model [25] (dashed line in Fig. 1e ) indicates that the charge-ordering fluctuations reach the size of a single unit cell roughly around T *. The survival of the optical spectral weight transfer W ( T ) up to this temperature implies that the mid-IR pseudogap is sensitive to charge correlations at a very localized scale in the Ni-O plane which—as illustrated in Fig. 1f —grow into patches of short-range charge order and finally into long-range charge stripes below T CO . Fano effect of the Ni-O stretch mode The sharp low-energy peak in σ 1 ( ω ) around 680 cm −1 is the Ni-O stretching mode [14] , which is further detailed in Fig. 2a (circles). As the crystal is cooled from room temperature to 30 K, this phonon resonance exhibits a strong blueshift of ≈15 cm −1 . Importantly, the lineshape becomes increasingly asymmetric at lower temperatures while it develops a broad low-energy tail. This distinct shape is characteristic of a Fano resonance, arising from quantum interference between the narrowband phonon resonance and the broadband electronic background [26] , [27] , [28] , [29] . Indeed, the phonon conductivity lineshape is well represented by the Fano model indicated by the lines in Fig. 2a , in which a constant electronic background has been subtracted (more details can be found in the Supplementary Methods ). Here is the reduced energy, where Г denotes the total linewidth and Ω ph the bare energy of the phonon. The asymmetry, and thus the interaction, is governed by the Fano parameter q. The temperature dependence of these parameters ( Fig. 2b–d ) shows that the Fano resonance develops without any sharp transition at T CO , instead evolving over a large temperature range at least comparable to T *. 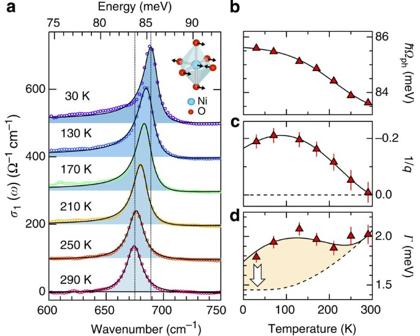Figure 2: Temperature-dependent electron–phonon coupling of the Ni-O stretch mode. (a) Optical conductivity around the Ni-O stretching mode (open circles), for different temperatures as indicated. Lines: fit with the Fano model explained in the text. Data are offset for clarity and the shaded area indicates the difference to a constant electronic background, which was removed by subtracting the conductivity at 800 cm−1. (b–d) Temperature dependence of the parameters from the Fano model fit (symbols) showing the mode frequencyΩph, the Fano parameter 1/qand the total linewidthГ, respectively. Solid lines: guide to the eye. Dashed line: anharmonic line broadening remaining after considering the Fano contribution (yellow area) derived from the ultrafast modulation (see text). Error bars represent the 95% confidence interval in extracting the fitting parameters and include possible uncertainties due to the background subtraction procedure (SeeSupplementary Methods). Figure 2: Temperature-dependent electron–phonon coupling of the Ni-O stretch mode. ( a ) Optical conductivity around the Ni-O stretching mode (open circles), for different temperatures as indicated. Lines: fit with the Fano model explained in the text. Data are offset for clarity and the shaded area indicates the difference to a constant electronic background, which was removed by subtracting the conductivity at 800 cm −1 . ( b – d ) Temperature dependence of the parameters from the Fano model fit (symbols) showing the mode frequency Ω ph , the Fano parameter 1/ q and the total linewidth Г , respectively. Solid lines: guide to the eye. Dashed line: anharmonic line broadening remaining after considering the Fano contribution (yellow area) derived from the ultrafast modulation (see text). Error bars represent the 95% confidence interval in extracting the fitting parameters and include possible uncertainties due to the background subtraction procedure (See Supplementary Methods ). Full size image Assuming a featureless electronic background, the inverse Fano parameter 1/ q ( Fig. 2c ) is directly proportional to the electron–phonon interaction strength V e-ph via the relation [26] , [27] , [28] . where σ el and σ ph are the conductivities of the electronic background and phonon transition, respectively. The large change of 1/ q indicates a dramatic increase in electron–phonon coupling V e-ph of the Ni-O stretching mode. This effect is particularly surprising, as it occurs despite the decrease in the low-energy electronic conductivity with lower temperatures. A mere reduction in screening cannot account for this observation because the Ni-O lineshape remains symmetric as the carrier density decreases with doping [13] . On the other hand, the electron–phonon interaction can sensitively depend on the spatial arrangement of holes along the interatomic bonds [4] , [30] . The picture that emerges is that the strong temperature-dependent changes in the mid-IR conductivity of LSNO track the increasing localization of charges around specific Ni sites upon cooling, resulting in a strongly enhanced coupling with in-plane Ni-O stretching vibrations. Such enhanced coupling can, in turn, stabilize both the on-site charge localization and stripe patterns as described theoretically [31] , [32] , [33] . Ultrafast dynamics of pseudogap and Fano effect To understand the interplay between these low-energy degrees of freedom in LSNO, we have investigated the ultrafast response of the mid-IR conductivity to femtosecond optical excitation. Pump pulses with 50-fs duration and 800 nm wavelength were employed to perturb the charge order via d–d and Ni-O charge excitations [15] , [22] , [34] , and changes of the in-plane mid-IR reflectivity were probed through ≈150-fs pulses broadly tunable from 80 meV to 1 eV. 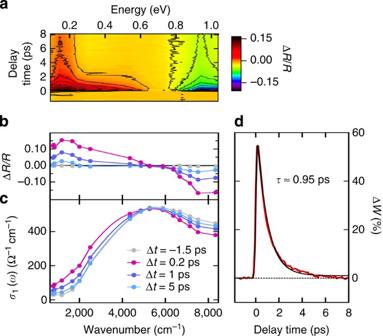Figure 3: Mid-infrared pseudogap dynamics. (a) Transient reflectivity variations ΔR/Ras a function of energy and time delay measured at 30 K and for 1 mJ cm−2absorbed pump fluence. Contour lines (black) are indicated in steps of 0.02. (b) Spectral cuts of photo-induced reflectivity variations ΔR/Rat representative time delays Δt, and (c) the resulting spectra of the transient conductivityσ1(ω,Δt). (d) Transient change ΔW(t) of the low-energy spectral weightW, normalized to its full-scale variation upon heating from 30 to 290 K. Solid line: exponential decay fit withτ=950 fs convoluted with the pulse temporal profile. Figure 3a shows the induced reflectivity changes Δ R ( ω ,Δ t )/ R ( ω ) at T =30 K, as a function of probe photon energy ħω and pump–probe delay time Δ t . Spectral cuts at specific delay times are indicated in Fig. 3b . After excitation, the reflectivity increases for photon energies below ≈0.65 eV, with a concurrent decrease above this pivotal energy. The reflectivity changes occur immediately, within the time resolution, and subsequently decay back towards equilibrium on a timescale of several hundreds of femtoseconds. The time evolution of the optical conductivity can be obtained from these data, as both the equilibrium conductivity and Δ R are characterized over a broad spectral range. The resulting transient conductivity spectra σ 1 ( ω ,Δ t ) in Fig. 3c reveal an increase in conductivity below ≈0.6 eV and a decrease above, clearly evidencing the ultrafast filling of the mid-IR pseudogap. The corresponding spectral weight dynamics in Fig. 3d shows the almost immediate (resolution-limited) recovery of ≈50% of the low-energy spectral weight lost upon cooling, reflecting a fast delocalization of holes that relaxes exponentially with τ =950 fs back to equilibrium. Figure 3: Mid-infrared pseudogap dynamics. ( a ) Transient reflectivity variations Δ R/R as a function of energy and time delay measured at 30 K and for 1 mJ cm −2 absorbed pump fluence. Contour lines (black) are indicated in steps of 0.02. ( b ) Spectral cuts of photo-induced reflectivity variations Δ R/R at representative time delays Δ t , and ( c ) the resulting spectra of the transient conductivity σ 1 ( ω ,Δ t ). ( d ) Transient change Δ W ( t ) of the low-energy spectral weight W , normalized to its full-scale variation upon heating from 30 to 290 K. Solid line: exponential decay fit with τ =950 fs convoluted with the pulse temporal profile. Full size image In turn, the dynamics of lattice distortions is measured in a similar manner but now tuning the probe wavelength across the Ni-O stretching mode resonance. The resulting conductivity spectra are shown in Fig. 4a . The peak frequency Ω max of the Ni-O mode (squares, Fig. 4b ) remains effectively unchanged after ultrafast excitation. For comparison, we plot the dynamics (solid line in Fig. 4b ) expected if the phonon mode and electronic spectral weight W ( T ) were instantaneously coupled — that is followed the dependence of Figs 1c and 2b with a common quasi-equilibrium temperature. The stark contrast underscores the non-thermal nature of the photoexcited phase and demonstrates that the Ni-O phonon hardening in equilibrium is decoupled from pseudogap physics, arising instead from anharmonic lattice effects and screening. This absence of a line shift also rules out a significant increase in the Ni-O phonon population or large photo-induced structural dynamics on the sub-picosecond timescale. 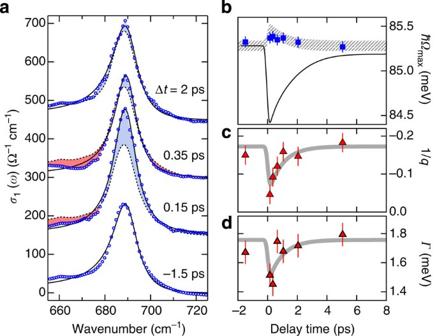Figure 4: Ultrafast suppression of electron–phonon coupling. (a) Non-equilibrium optical conductivity around the Ni-O stretching mode (circles) at representative delay times after photoexcitation at 30 K and for 1 mJ cm−2absorbed pump fluence. Dashed lines: equilibrium conductivity, solid lines: Fano model. Blue and red shaded regions indicate a transient increase or decrease, respectively, of the conductivity. (b) Dynamics of the Ni-O mode peak energyΩmax(squares), compared with that expected for direct coupling between the electronic spectral weight and equilibrium phonon shift as explained in the text (solid line). Hatched area: transient peak energyΩmax(t)=Г(t)/q(t)+Ωph(T=30 K) expected from the Fano model, taking into account the fits in panels (c,d) and their corresponding uncertainties (95% confidence interval). (c,d) Dynamics of the Fano coupling parameter 1/qand the phonon linewidthГ(symbols), along with model curves (thick lines) with a single-exponential decay time fixed toτ=950 fs as obtained from the spectral weight dynamics inFig. 3d. Error bars represent the 95% confidence interval in extracting the fitting parameters and include possible uncertainties because of the background subtraction procedure (SeeSupplementary Methods). Figure 4: Ultrafast suppression of electron–phonon coupling. ( a ) Non-equilibrium optical conductivity around the Ni-O stretching mode (circles) at representative delay times after photoexcitation at 30 K and for 1 mJ cm −2 absorbed pump fluence. Dashed lines: equilibrium conductivity, solid lines: Fano model. Blue and red shaded regions indicate a transient increase or decrease, respectively, of the conductivity. ( b ) Dynamics of the Ni-O mode peak energy Ω max (squares), compared with that expected for direct coupling between the electronic spectral weight and equilibrium phonon shift as explained in the text (solid line). Hatched area: transient peak energy Ω max ( t )= Г ( t )/ q ( t )+ Ω ph ( T =30 K) expected from the Fano model, taking into account the fits in panels ( c , d ) and their corresponding uncertainties (95% confidence interval). ( c , d ) Dynamics of the Fano coupling parameter 1/ q and the phonon linewidth Г (symbols), along with model curves (thick lines) with a single-exponential decay time fixed to τ =950 fs as obtained from the spectral weight dynamics in Fig. 3d . Error bars represent the 95% confidence interval in extracting the fitting parameters and include possible uncertainties because of the background subtraction procedure (See Supplementary Methods ). Full size image In contrast, the transient shape of the Ni-O stretching mode in Fig. 4a is strongly affected by photoexcitation. A decrease in conductivity occurs in the low-energy wing concurrent with a large increase in the conductivity at the phonon peak. This corresponds to an almost complete ultrafast suppression of the Fano effect, and thus of the electron–phonon coupling. The time-dependent parameters obtained from the Fano fits are plotted in Fig. 4c,d , showing the temporary decrease in 1/ q and the linewidth. Their recovery is compatible with the spectral weight decay time as indicated by the model curves (thick lines). The resulting Fano-induced shift of the resonance peak Ω max ( t ) in Fig. 4b (hatched line) is small and compatible with the observations. The photo-induced narrowing of the lattice resonance ( Fig. 4d ) further confirms the temporarily reduced electron–phonon interactions. From this, one can estimate the broadening attributable to the coupling (arrow, Fig. 2d ), with the remaining linewidth modeled by multiphonon anharmonic processes (dashed line) [29] . The rapid suppression of the Ni-O Fano effect, whose recovery tracks the electronic spectral weight, suggests a strong dependence of the electron–phonon coupling on the degree of charge localization. This localized coupling can stabilize the ground state, yet it is unlikely the driving force of the relaxation dynamics, as a time-varying coupling parameter should result in a highly non-exponential, accelerating recovery of W ( t ) that is not observed. The observed timescale can involve both electronic localization dynamics as observed in 1D Mott insulators [35] and coupling to the lattice heat bath. We note that the correlation between charge localization and enhanced electron–phonon coupling in our study is inferred not only from the concurrent dynamics but also from the temperature dependence of the equilibrium optical conductivity. This correspondence would be further strengthened by confirming the synchronous dynamics at additional excitation fluences below the present value (1 mJ cm −2 ), which are inaccessible in our experiment because of signal-to-noise limitations. Future studies with high-repetition rate laser sources will allow unravelling the dependence in the low-fluence regime. The ultrafast mid-IR response of LSNO can be compared to our recent time-resolved resonant XRD experiments, which measured the dynamics of the long-range stripe order parameter [22] . The mid-IR dynamics is significantly faster, with an initial ≈950-fs decay compared with the multi-picosecond recovery times of stripes at similar excitation levels. Charge localization and electron–phonon coupling thus represents the early dynamics of symmetry breaking, which precedes the slower recovery of long-range charge order at these fluences. Our observations clarify the role of the pseudogap phase below T * as a precursor that ultimately enables the organization of localized holes into stripe patterns at low temperatures. Notably, the nickelate pseudogap formation time observed here closely matches the ≈700-fs pseudogap dynamics in YBa 2 Cu 3 O 7- δ (ref. 18 ). Moreover, similarities with the cuprate pseudogap in momentum space were found in the highly doped metallic phase of LSNO governed by checkerboard charge fluctuations [16] . This opens intriguing perspectives on the pseudogap in correlated oxides and motivates further studies to explore dynamic interactions of real-space charge fluctuations and their roles in the formation of long-range order. The possibility to control charge localization and the electron–phonon coupling on ultrafast timescales can also lead to fascinating opportunities in the growing field of ultrafast oxide electronics [36] , [37] , [38] . Samples La 1.75 Sr 0.25 NiO 4 (LSNO) single crystals were grown using the floating zone method. The crystals were first oriented using Laue diffraction and cut along the [100] surface. We use orthorhombic notation to express the crystal structure, with [100] oriented 45° to the Ni-O bond direction within the ab plane. The LSNO crystal surface was optically polished for the experiments. The phase-transition temperature for the long-range charge order is ≈105 K and the spin-order transition occurs at slightly lower temperature below around ≈90 K. X-ray diffraction experiments X-Ray diffraction experiments were performed at the Advanced Light Source synchrotron, some results of which were reported in Lee et al . [22] . The X-ray absorption spectrum (XAS) near the Ni L 3 -edge was first measured to calibrate the incident photon energy. Then, the resonant diffraction experiments were performed on the charge-order peak, with the X-ray photon energy tuned to the Ni L 3 -edge at 851 eV. The diffraction signal of the CO reflection peak (0.554,0,1) at temperatures above T CO is shown in the Supplementary Fig. S1 along with corresponding fits using a squared-Lorentzian function. The peak intensity I and the correlation length ξ obtained from the fit coefficients (amplitude and full width at half maximum, FWHM, w ) are plotted in Fig. 1 of the main text. The correlation length is calculated using the equation , with the lattice spacing in the ab plane being a =5.41 Å and w being the FWHM expressed in reciprocal lattice units (r.l.u.). Mid-IR pump–probe experiments Pump–probe reflectivity measurements are performed using a Ti:sapphire femtosecond laser amplifier operating at 1 kHz repetition rate (Femtolasers Compact Pro), which generates pulses of 28-fs duration at λ =800 nm centre wavelength. Pump pulses are obtained by splitting off a fraction of the laser output, whereas the mid-IR and near-infrared (near-IR) probe pulses are generated via optical parametric amplification (0.5–1 eV tuning range) and cascaded difference frequency mixing of the near-IR signal and idler pulses in GaSe (≈80–400 meV range). The pump beam is oriented at normal incidence—that is, parallel to the [100] direction—whereas the probe angle of incidence is <10°. Pump and probe polarizations are oriented within the ab plane of the LSNO crystal. Average pump and probe spot sizes are d pump ≈400±50 and d probe ≈220±20 μm, respectively. Spot sizes are carefully calibrated at each wavelength through pinhole transmission measurements. The probe-to-pump intensity ratio is kept <1:10. High-precision single-shot detection is performed to sensitively measure the transient reflectivity changes as a function of the delay time between the pump and probe pulses. For this, the reflected probe energy was normalized to that of a reference pulse for each laser shot, as recorded with LN 2 -cooled HgCdTe detectors using gated integration. The time zero and pulse profiles are characterized at each wavelength through transient reflectivity pump–probe measurements of photoexcited carriers in a thin GaAs crystal. The pulse duration of the probe pulses is typically 150 fs. The probe beam is monochromatized after interaction with the sample using a mid-IR grating spectrometer (Acton SpectraPro 2300i). This allows us to substantially improve the spectral resolution without affecting the temporal resolution of the measurement. To allow for studies of the Ni-O stretching mode, the spectral resolution in the 700 cm −1 range was set to better than 2 cm −1 . In order to optimize the reproducibility of the spectral information, the data of the Ni-O stretching mode dynamics are acquired with a continuous scan of the spectrum at a set of fixed delay times. For this purpose, a single mid-IR pulse is used to span the range of interest, from 650 to 800 cm −1 . Standard pump–probe scans of the delay time at fixed wavelength are also used in this range to verify the accuracy of the time-domain information. Equilibrium optical conductivity Fourier-transform infrared (FTIR) spectroscopy measurements of the equilibrium reflectivity R ( ω ) were performed with a Bruker 66v/S vacuum FTIR spectrometer at Beamline 1.4.2 of the Advanced Light Source synchrotron. We employed a reflection geometry setup with 11° angle of incidence and a liquid helium optical cryostat equipped with KBr windows. A smooth continuation outside the experimental range is obtained from known optical data of similar samples [12] , [15] . To extract the optical conductivity σ( ω ) from the measured reflectivity data, we performed a Kramers–Kronig constrained variational fitting procedure. This procedure is inspired by the work of Kuzmenko [25] , and it is extended here to the case of non-equilibrium data as described further below. Following the original approach of Kuzmenko [24] , reflectivity data are first modeled with a standard multioscillator model of the complex dielectric function, ε mod ( ω ), which reproduces the main features of the data. Second, the addition of a small variational part, ε var ( ω ) to the total dielectric function, , allows the precise fitting of the fine details of the experimental data. ε var ( ω ) is calculated as a sum of N local contributions , where each ε i ( ω ) contribution is centred at the corresponding anchor point ω i and obeys the Kramers–Kronig transform. A function ε i ( ω ) with triangular shape in its imaginary part is the most effective in representing the local spectral weight contribution, with the real and imaginary parts [24] : with . The optical conductivity σ ( ω ) and reflectivity R ( ω ) can be readily calculated from ε ( ω ). The A i parameters are adjusted through the fitting procedure to best reproduce the measured reflectivity, thus determining ε ( ω ) and σ ( ω ). Transient optical conductivity In the experiments, we measure the transient reflectivity change Δ R ( ω ) of the photoexcited sample in a broad range of photon energies. The above variational model is expanded to calculate the corresponding conductivity change Δ σ ( ω ) in the photoexcited sample. For this, the photoexcited dielectric function ε exc ( ω ) is calculated as a sum of a variational dielectric function Δ ε ( ω ) and the equilibrium one, The variational part Δ ε is then optimized through a fitting procedure to best reproduce the measured excited-state reflectivity R exc ( ω )=Δ R ( ω )+ R ( ω ). The effect because of a frequency-dependent mismatch in penetration depths between pump and probe needs to be taken into account, as the photoexcited volume (penetration depth δ pump ≈150 nm at λ =800 nm) is generally a fraction of the probe volume ( δ probe ≈550 nm at λ =5 μm). The penetration depth is calculated through the standard formula and the full spectral dependence is shown in the Supplementary Fig. S2 . We considered an excited volume with exponentially decaying dielectric function change along the z direction. This problem was solved with a transfer matrix numerical calculation of the coherent reflection and transmission of a multilayer structure with up to 1,000 layers to approximate the smooth exponentially decaying changes. The results of this calculation are closely reproduced with a less numerically intensive method, where the photoexcited volume is approximated with a single thin-film layer on top of a substrate with equilibrium optical properties. In this case, however, coherent artifacts arising from multiple reflections at the film–substrate interface must be avoided. This is achieved in the simulation by integrating over a spread of film thicknesses of ≈50%. After confirming the consistency with the transfer matrix method, this approach was employed to extract the optical conductivity changes over a large number of frequency and time steps. How to cite this article: Coslovich, G. et al . Ultrafast charge localization in a stripe-phase nickelate. Nat. Commun. 4:2643 doi: 10.1038/ncomms3643 (2013).